Sam68 modulates the promoter specificity of NF-κB and mediates expression of CD25 in activated T cells CD25, the alpha chain of the interleukin-2 receptor, is expressed in activated T cells and has a significant role in autoimmune disease and tumorigenesis; however, the mechanisms regulating transcription of CD25 remain elusive. Here we identify the Src-associated substrate during mitosis of 68 kDa (Sam68) as a novel non-Rel component in the nuclear factor-kappaB (NF-κB) complex that confers CD25 transcription. Our results demonstrate that Sam68 has an essential role in the induction and maintenance of CD25 in T cells. T-cell receptor engagement triggers translocation of the inhibitor of NF-κB kinase alpha (IKKα) from the cytoplasm to the nucleus, where it phosphorylates Sam68, causing complex formation with NF-κB in the nucleus. These findings reveal the important roles of KH domain-containing components and their spatial interactions with IKKs in determining the binding targets of NF-κB complexes, thus shedding novel insights into the regulatory specificity of NF-κB. CD25, the alpha chain of interleukin-2 receptor (IL-2R), is inducibly expressed and required for formation of the high-affinity IL-2R. Elevated expression of CD25 has been detected in T cells in an array of autoimmune diseases, allograft rejection and lymphoid neoplasms [1] , and a large variety of cancers [2] . Moreover, soluble CD25 shed from the cell surface has been proposed as a prognostic indicator in cancer patients, with high plasma levels correlating with poor survival rates [2] . It is well known that the promoter in the CD25 gene contains multiple DNA regulatory elements that bind to key transcription factors, in particular, nuclear factor-kappaB (NF-κB) and nuclear factor of activated T cells (NF-AT); however, the mechanism(s) governing the specific transcription of CD25 in normal and tumour cells remain elusive. Diverse stimuli can activate NF-κB and induce an ever-increasing list of target genes, which involve manifold biological activities [3] , [4] , [5] , [6] . NF-κB binds 10 nucleotide cognate sites called κB sites that appear to be a minimal requirement for regulation, but insufficient for gene induction [7] , [8] . It is still a long-standing question how NF-κB selectively recognizes a small subset of relevant κB sites from the large excess of potential binding sites [6] . Furthermore, the molecular size and affinity of the native NF-κB complex are of greater magnitude than can be accounted for by reconstituted heterodimers of Rel proteins [9] , [10] . Beyond the Rel components, we recently identified ribosomal protein S3 (RPS3) as an integral and functional component in NF-κB complexes [7] . RPS3 appears to select particular genomic κB sites to be activated and preferentially directs high-affinity binding to κB sites with certain sequence specificities, therefore serving as a ‘specifier’ subunit of NF-κB [7] . The identification of RPS3 suggested a new mechanism in which DNA-binding activity could be regulated within NF-κB complexes by the synergistic interactions between Rel and non-Rel components [7] , [8] . Moreover, the significance of RPS3-dependent specific NF-κB transcription has been highlighted in an increasing number of key pathophysiological processes [7] , [11] , [12] , [13] , [14] , [15] , [16] , [17] , [18] . However, the full regulatory spectra of NF-κB cannot be fully explained by the inclusion of RPS3. There are conditions in which NF-κB accumulates in the nucleus, while there is no CD25 expression, implying that NF-κB is necessary but not sufficient for CD25 induction [2] . In particular, CD25 is among those NF-κB target genes whose transcription does not require RPS3 during T-cell activation [7] . Given its critical role in autoimmune diseases and diverse malignancies, deciphering the NF-κB-mediated specific transcription of CD25 will better our understanding of the regulatory specificity of NF-κB and elucidate novel target molecules for pharmacological interventions. Sam68 (Src-associated substrate during mitosis of 68 kDa) belongs to the heteronuclear ribonucleoprotein particle K (hnRNP K) homology (KH) domain family of RNA-binding proteins [19] , [20] . Sam68 is versatile protein functioning in a variety of cellular processes, ranging from regulating RNA stability, RNA alternative splicing, adipogenesis, spermatogenesis, carcinogenesis and others [19] , [20] , [21] , [22] , [23] , [24] , [25] , [26] , [27] , [28] , [29] . Emerging evidence suggests Sam68 functions as a signalling molecule in multiple signalling pathways [30] , in particular a recently revealed role of Sam68 in both NF-κB activation and apoptosis initiated through the TNF receptor [31] . However, it remains largely unknown whether Sam68, as a preferentially nuclear protein, has an important role in signal transduction and gene regulation in the nucleus, in spite of its emerging role in regulating transcriptional activity implicated by recent studies [32] , [33] , [34] . Here we identify Sam68 as a novel DNA-binding component that is critical for NF-κB to specifically recognize the CD25 κB site. T-cell receptor (TCR) engagement triggered the inhibitor of NF-κB kinase alpha (IKKα) to translocate from the cytoplasm to the nucleus, where it phosphorylated Sam68. Phosphorylated Sam68 associated with nuclearly translocated NF-κB complexes, and facilitated binding to the CD25 κB site for full gene induction. Our results demonstrate there can be at least two biochemically distinct p65-p50 NF-κB complexes in the nucleus of the same cells at the same time, reinforcing the notion that NF-κB consists of both Rel and non-Rel subunits that actually comprise multiple protein complexes with different gene activation specificities. Recognition of CD25 κB DNA by NF-κB does not depend on RPS3 We recently identified RPS3 as non-Rel component of NF-κB that targets the NF-κB DNA-binding complex to certain κB motifs [7] . To examine whether RPS3 is required for recruiting the NF-κB complex to target genes during T-cell activation, we performed chromatin immunoprecipitation (ChIP) to analyse endogenous p65 recruitment to the promoters of known NF-κB target genes CD25 , IL8 and NFKBIA [35] , [36] , [37] . Knockdown of RPS3 by small interfering RNAs (siRNA) remarkably attenuated the TCR stimulation-induced p65 recruitment to the κB regions of NFKBIA and IL8 promoters [7] ( Fig. 1a ). The p65 enrichment was specific, as there was negligible recruitment of p65 to the ACTB promoter that does not contain any κB sites ( Fig. 1a ). By contrast, the transcription and the recruitment of p65 to the CD25 κB site was undiminished and perhaps even slightly augmented [7] ( Fig. 1a ). Moreover, ablation of RPS3 specifically abolished the TCR stimulation-induced NF-κB gel shift complex formed with NFKBIA κB probe ( Fig. 1b , compare lanes 2 and 4), without affecting the complex formed with CD25 κB probe ( Fig. 1c , compare lanes 6 and 8). These data suggest that RPS3 is not required for NF-κB to form a stable complex with CD25 κB DNA. We performed supershift assays and determined that both p65 and p50 exist in the CD25 κB DNA-binding complex ( Fig. 1c , lanes 10 and 11). Of note, the migration of the complexes formed with the NFKBIA κB site and the CD25 κB site opens up the possibility that they have different biochemical compositions ( Fig. 1b ). Furthermore, heterodimers formed by recombinant p65 and p50 bind poorly, whereas the nuclear extracts from NF-κB constitutively activated HUT102 lymphoma cells exhibit high affinity to CD25 κB DNA ( Fig. 1d , lanes 12 and 13). These data suggest that Rel components are not sufficient for the high affinity to CD25 κB DNA. Therefore, at least one other RPS3-like ‘specifier’ component in the NF-κB complex could confer the recognition of CD25 κB DNA. 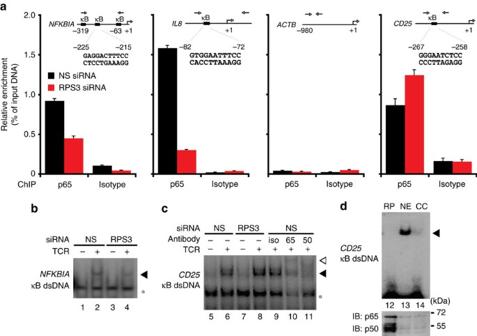Figure 1: Recognition ofCD25κB DNA requires Rel components but does not depend on RPS3. (a) Jurkat cells transfected with nonspecific (NS) or RPS3 siRNAs were stimulated with αCD3/CD28 (1 μg ml−1each). The recruitment of endogenous p65 to the promoters ofNFKBIA,IL8,ACTB, andCD25genes were analysed by ChIP with either isotype or p65 antibodies. Diagrams inside show the sequences and locations of κB sites in corresponding promoters. The p65-bound DNA was analysed by quantitative real-time PCR (primers, above diagrammed) and normalized to input DNA (mean±s.d.,n=3). (b,c) Jurkat cells were left untreated (−) or stimulated (+) as ina, after transfection with siRNAs. The nuclear extracts were analysed by EMSA with a32P-labelledNFKBIAκB probe (b) orCD25κB probe (c). The nonspecific bands and corresponding κB DNA complexes were labelled with asterisks and arrowheads, respectively. Inc, the supershiftCD25κB bands by isotype (iso), p65 (65), or p50 (50) antibodies were labelled with an open arrowhead. (d) Recombinant p65 and p50 proteins (RP) or nuclear extracts (NE) from HUT102 cells was subjected to an EMSA with a32P-labelledCD25κB double-stranded DNA, in some cases with 100-fold unlabeledCD25κB oligonucleotide competitor (CC). TheCD25κB site-specific NF-κB DNA-binding complex is labelled with a triangle. The amount of p65 and p50 proteins in recombinant proteins and nuclear extracts were immunoblotted (IB) with indicated antibodies. Figure 1: Recognition of CD25 κB DNA requires Rel components but does not depend on RPS3. ( a ) Jurkat cells transfected with nonspecific (NS) or RPS3 siRNAs were stimulated with αCD3/CD28 (1 μg ml −1 each). The recruitment of endogenous p65 to the promoters of NFKBIA , IL8 , ACTB , and CD25 genes were analysed by ChIP with either isotype or p65 antibodies. Diagrams inside show the sequences and locations of κB sites in corresponding promoters. The p65-bound DNA was analysed by quantitative real-time PCR (primers, above diagrammed) and normalized to input DNA (mean±s.d., n =3). ( b , c ) Jurkat cells were left untreated (−) or stimulated (+) as in a , after transfection with siRNAs. The nuclear extracts were analysed by EMSA with a 32 P-labelled NFKBIA κB probe ( b ) or CD25 κB probe ( c ). The nonspecific bands and corresponding κB DNA complexes were labelled with asterisks and arrowheads, respectively. In c , the supershift CD25 κB bands by isotype (iso), p65 (65), or p50 (50) antibodies were labelled with an open arrowhead. ( d ) Recombinant p65 and p50 proteins (RP) or nuclear extracts (NE) from HUT102 cells was subjected to an EMSA with a 32 P-labelled CD25 κB double-stranded DNA, in some cases with 100-fold unlabeled CD25 κB oligonucleotide competitor (CC). The CD25 κB site-specific NF-κB DNA-binding complex is labelled with a triangle. The amount of p65 and p50 proteins in recombinant proteins and nuclear extracts were immunoblotted (IB) with indicated antibodies. Full size image Sam68 is associated with the CD25 κB DNA-binding complex To explore this possibility, we utilized the human T-lymphotropic virus type I (HTLV-I)-carrying T-cell lymphoma cell line HUT102, where the NF-κB signalling and CD25 expression are constitutively activated [38] ( Figs 1d and 2a ). We hypothesized the NF-κB complex binding to CD25 κB DNA could contain other KH domain proteins, as KH domains can bind both proteins and nucleic acids and therefore can potentially serve as a platform facilitating protein/protein–protein/DNA interaction [39] , and they have been illustrated as essential functional components of several transcriptional complexes [40] . To evaluate this hypothesis, we immunoprecipitated p65 from nuclear extracts derived from HUT102 cells and screened the immunoprecipitate with antibodies against various KH domain proteins ( Table 1 ). RPS3 was shown to interact strongly with p65 ( Table 1 ), indicating the active transcription of some RPS3-dependent genes in HUT102 cells. In support of this notion, the IL2 gene, whose transcription requires RPS3 (ref. 7 ), is consistently activated by NF-κB in HUT102 cells [38] . Interestingly, Sam68, another KH domain protein with remarkable nucleic acid-binding capability [41] , [42] , exhibited strong interaction with p65 ( Table 1 , Fig. 2b ). Moreover, the specific Sam68–p65 interaction was verified by a pull-down assay using GST-tagged Sam68 and HUT102 cell nuclear extracts ( Supplementary Fig. S1 ). 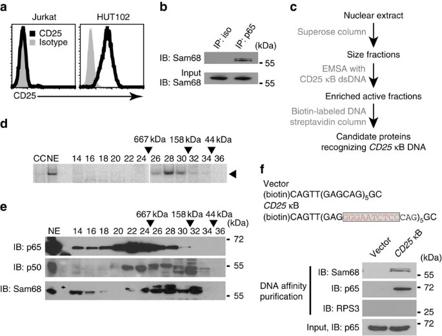Figure 2: Sam68 is a novel p65-interacting protein in the NF-κB complex binding to theCD25κB site. (a) The cell surface CD25 expression in resting Jurkat A3 cells and HUT102 cells was stained with isotype antibody or PE-conjugated CD25 antibody, and analysed by FACS. (b) Nuclear extracts from HUT102 cells were immunoblotted (IB) directly or after immunoprecipitation (IP) with isotype (iso) or p65 antibody for Sam68. (c) The purification scheme for proteins specifically recognizingCD25κB DNA by gel filtration and DNA affinity purification in the HUT102 cells. (d) Nuclear extracts prepared from HUT102 cells were separated on a Superose 6 gel filtration column. The fractions 14–36 were interrogated forCD25κB DNA-binding activity in EMSAs. The unfractionated nuclear extract (NE) was also analysed with32P-labelledCD25κB probe or with 100-fold unlabelledCD25κB oligonucleotide competitors (CC). TheCD25κB complex was indicated by a triangle and the elution positions of protein standards are indicated. (e) The Superose 6 fractions 14–36 were immunoblotted (IB) with p65, p50, and Sam68 antibodies and the elution positions of protein standards are indicated. NE indicates the unfractionated nuclear extract. (f) Schematic diagram of vector double-stranded DNA or that contains five copies ofCD25κB sites. Immunoblot (IB) of the elution after DNA affinity purification for indicated proteins from pooled fractions from 24 to 30 harboring highCD25κB DNA-binding activity. Figure 2: Sam68 is a novel p65-interacting protein in the NF-κB complex binding to the CD25 κB site. ( a ) The cell surface CD25 expression in resting Jurkat A3 cells and HUT102 cells was stained with isotype antibody or PE-conjugated CD25 antibody, and analysed by FACS. ( b ) Nuclear extracts from HUT102 cells were immunoblotted (IB) directly or after immunoprecipitation (IP) with isotype (iso) or p65 antibody for Sam68. ( c ) The purification scheme for proteins specifically recognizing CD25 κB DNA by gel filtration and DNA affinity purification in the HUT102 cells. ( d ) Nuclear extracts prepared from HUT102 cells were separated on a Superose 6 gel filtration column. The fractions 14–36 were interrogated for CD25 κB DNA-binding activity in EMSAs. The unfractionated nuclear extract (NE) was also analysed with 32 P-labelled CD25 κB probe or with 100-fold unlabelled CD25 κB oligonucleotide competitors (CC). The CD25 κB complex was indicated by a triangle and the elution positions of protein standards are indicated. ( e ) The Superose 6 fractions 14–36 were immunoblotted (IB) with p65, p50, and Sam68 antibodies and the elution positions of protein standards are indicated. NE indicates the unfractionated nuclear extract. ( f ) Schematic diagram of vector double-stranded DNA or that contains five copies of CD25 κB sites. Immunoblot (IB) of the elution after DNA affinity purification for indicated proteins from pooled fractions from 24 to 30 harboring high CD25 κB DNA-binding activity. Full size image Table 1 Interactions of selected KH domain-containing proteins with p65 in HUT102 cells Full size table To examine whether Sam68 is a protein component that determines the recognition of CD25 κB DNA by NF-κB, we separated the nuclear extracts from HUT102 cells into sequential fractions. The CD25 κB DNA-binding active fractions were collected for a subsequent DNA affinity purification to separate the potential binding protein(s) ( Fig. 2c ). Unexpectedly, the peaks of the CD25 κB DNA-binding activities in the sequential nuclear fractions through gel filtration ( Fig. 2d ) did not coincide with the distribution peaks of neither p65 nor p50 in the fractions ( Fig. 2e ), suggesting that the p65 or p50 is not the limiting factor for NF-κB to bind the CD25 κB site as long believed. In contrast, the distribution of Sam68 better approximated the CD25 κB DNA-binding activities ( Fig. 2e ), which hints that Sam68 could be a prerequisite for NF-κB recognizing the CD25 κB DNA. We then isolated the putative candidate(s) conferring NF-κB-binding specificity to the CD25 κB site by DNA affinity purification using the enriched active fractions (26–30 in Fig. 2d ). Both p65 and Sam68 were enriched in the affinity eluate from biotin-labelled double-stranded DNA containing five copies of CD25 κB sites but not in the control DNA ( Fig. 2f ). RPS3 was not observed in the NF-κB complex binding to the CD25 κB DNA ( Fig. 2f ), independently demonstrating that RPS3 is not required for NF-κB binding to the CD25 κB site [7] , despite the fact that abundant RPS3 was present in the nucleus and associated with p65 ( Table 1 ). These results suggest that Sam68 could be an integral component of NF-κB DNA-binding complex to the CD25 κB site. Sam68 is an integral component in the CD25 NF-κB complex Provided that Sam68 preferentially localizes in the nucleus ( Supplementary Fig. S2 ) [19] , we first performed ChIP assays to examine whether Sam68 could be recruited to the CD25 promoter. We found precipitation of either p65 or Sam68, but not isotype control, gave almost identical signal for the 200–300 base-pair CD25 promoter region containing κB sites, in HUT102 cells ( Fig. 3a ). In contrast, neither Sam68 nor p65 gave a significant enrichment signal for the ACTB promoter that lacks κB sites ( Fig. 3a ). These results suggest that Sam68 could be a component of the NF-κB complex formed at the CD25 κB site, which validates, in intact nuclear chromatin, our biochemical observation that both Sam68 and p65 were co-enriched in the affinity purification eluate using CD25 κB DNA ( Fig. 2f ). 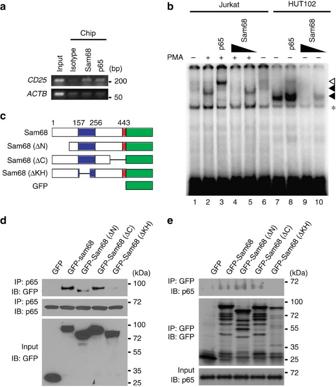Figure 3: Sam68 is an integral component in the NF-κB complex binding to theCD25κB site. (a) HUT102 cells were used for ChIP assays with indicated antibodies. The recruitment of indicated proteins to the κB region ofCD25promoter orACTBpromoter in the immunoprecipitates was detected by PCR. (b) Nuclear extracts of HUT102 cells (lanes 7–10) and Jurkat cells (lanes 1–6) treated with (+) or without (−) PMA (50 ng ml−1, 30 min) were analysed by EMSA with32P-labelledCD25κB oligonucleotides. Supershift analysis was conducted with p65 or different doses of Sam68 antibodies (lanes 3–5 and 8–10).CD25κB DNA-binding complexes in Jurkat cells and HUT102 cells are labelled with filled triangles, and the supershifted bands and nonspecific bands are labelled with an open triangle and an asterisk, respectively. (c) Schematic diagram of the full-length and truncated mutants (ΔN lacks residues 1–102, ΔC lacks residues 347−443, and ΔKH lacks residues 165–224) of Sam68 fused with EGFP. The hnRNP K homology (KH) domain (residues 157–256) and NLS are labelled in blue and red, respectively. (d,e) Whole-cell lysates from HEK293T cells transfected with GFP vehicle or indicated GFP-fused full-length or truncated Sam68, were immunoblotted (IB) directly or after immunoprecipitation (IP) with p65 antibody (d) or GFP antibody (e) for indicated proteins. Figure 3: Sam68 is an integral component in the NF-κB complex binding to the CD25 κB site. ( a ) HUT102 cells were used for ChIP assays with indicated antibodies. The recruitment of indicated proteins to the κB region of CD25 promoter or ACTB promoter in the immunoprecipitates was detected by PCR. ( b ) Nuclear extracts of HUT102 cells (lanes 7–10) and Jurkat cells (lanes 1–6) treated with (+) or without (−) PMA (50 ng ml −1 , 30 min) were analysed by EMSA with 32 P-labelled CD25 κB oligonucleotides. Supershift analysis was conducted with p65 or different doses of Sam68 antibodies (lanes 3–5 and 8–10). CD25 κB DNA-binding complexes in Jurkat cells and HUT102 cells are labelled with filled triangles, and the supershifted bands and nonspecific bands are labelled with an open triangle and an asterisk, respectively. ( c ) Schematic diagram of the full-length and truncated mutants (ΔN lacks residues 1–102, ΔC lacks residues 347−443, and ΔKH lacks residues 165–224) of Sam68 fused with EGFP. The hnRNP K homology (KH) domain (residues 157–256) and NLS are labelled in blue and red, respectively. ( d , e ) Whole-cell lysates from HEK293T cells transfected with GFP vehicle or indicated GFP-fused full-length or truncated Sam68, were immunoblotted (IB) directly or after immunoprecipitation (IP) with p65 antibody ( d ) or GFP antibody ( e ) for indicated proteins. Full size image To determine whether Sam68 is incorporated into the NF-κB DNA-binding complex, we utilized electrophoretic mobility shift assays (EMSAs) with nuclear extracts derived from either resting or stimulated Jurkat cells. PMA stimulation strongly induced formation of an NF-κB band as probed by CD25 κB oligonucleotides ( Fig. 3b , compare lanes 1 and 2). The specificity of the band was confirmed by cold oligonucleotide competition: CD25 κB oligonucleotides competed away, whereas OCT1 oligonucleotides did not diminish, the induced band ( Supplementary Fig. S3 ). The addition of p65 antibody indicated that the induced band contains the NF-κB p65 subunit ( Fig. 3b , lane 3), consistent with previous reports [7] . More importantly, Sam68 antibody blocked the formation of CD25 κB DNA-binding complexes, in a dose-dependent manner ( Fig. 3b , lanes 4 and 5), verifying that endogenous Sam68 is an integral component for the NF-κB complex that forms with the CD25 κB oligonucleotides. A similar result was obtained in nuclear extracts from HUT102 cells, where CD25 is constitutively activated through NF-κB ( Fig. 3b , lanes 7–10). Of note, the distinct migration of PMA-induced CD25 κB DNA-binding complex in Jurkat cells and constitutively activated CD25 κB DNA-binding complex in HUT102 cells ( Fig. 3b , compare lanes 2 and 7), suggests again that other component(s) beyond Rel subunits complex with the CD25 κB DNA and at least Sam68 is one of such protein(s). The notion that Sam68 and p65 could be jointly recruited as an NF-κB complex to the CD25 κB site was further supported by a structure–function study ( Figs. 3c–e , Supplementary Fig. S4 ). Using various truncations of Sam68, we sought to understand the key domain(s) in Sam68 for its interaction with p65. We detected the association of full-length, ΔN, and ΔC truncated Sam68 to p65, but not GFP vehicle ( Fig. 3d ). In contrast, deletion of the essential core of KH domain (amino acids (a.a.) 165–224) of Sam68 abolished the Sam68–p65 association ( Fig. 3d ). In a reverse immunoprecipitation, we obtained similar results ( Fig. 3e ), thus confirming the KH domain of Sam68 is required for p65 binding. The corresponding analysis of p65 revealed the Rel homologue domain (a.a. 1–311) was necessary, whereas neither the N-terminal portion nor the dimerization domain of p65 was sufficient for Sam68 binding ( Supplementary Fig. S4 ). The Rel homologue domain of p65 and the KH domain of Sam68 both possess nucleic acid-binding capabilities, thus Sam68 could regulate the binding of NF-κB complexes to CD25 κB DNA. Sam68 is critical for CD25 gene transcription To evaluate the role of Sam68 in NF-κB-mediated CD25 gene transcription, we examined luciferase reporter genes in Jurkat cells following Sam68 knockdown. Corresponding to the knockdown efficiency ( Fig. 4a ), Sam68 silencing dramatically attenuated p65 overexpression-induced luciferase reporter expression driven by a CD25 κB promoter ( Fig. 4b ). By contrast, knockdown of Sam68 did not decrease the induced expression of a luciferase reporter driven by either the activator protein 1 (AP-1) or NF-AT promoter ( Supplementary Fig. S5 ). Moreover, Sam68 knockdown remarkably attenuated the CD25 mRNA levels in Jurkat cells stimulated with PMA plus ionomycin (PMA/I) ( Fig. 4c ) and HUT102 cells ( Supplementary Fig. S6 ). Taken together, these data indicate a specific role of Sam68 in CD25 transcription. 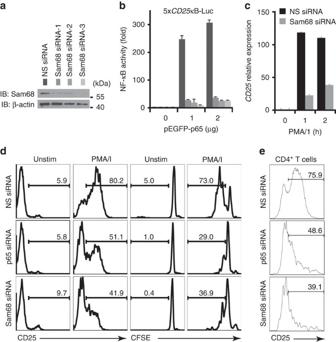Figure 4: The critical role of Sam68 in the expression of theCD25gene in T cells. (a) Jurkat cells were transfected with nonspecific (NS) or three different Sam68-specific siRNAs. After 72 h, the knockdown of Sam68 was examined by immunoblot (IB) for Sam68 with β-actin as a loading control. (b) NF-κB luciferase assay (mean±s.d.,n=3) of Jurkat cells transfected with nonspecific (NS) or Sam68 siRNAs, together with indicated amount of p65 plasmids and a luciferase reporter gene driven by 5 ×CD25κB sites. (c) Real-time PCR quantization (mean±s.d.,n=3) of mRNA level ofCD25normalized toGAPDHin Jurkat cells silenced with NS or pooled Sam68 siRNAs and stimulated by 50 ng ml−1PMA plus 1.5 μM ionomycin (PMA/I) for indicated time. (d) Human peripheral blood T lymphocytes were transfected with nonspecific (NS), p65, or Sam68 siRNAs and then stimulated with PMA/I or left unstimulated (Unstim). Flow cytometry histograms of T cells with CD25 induction and carboxyfluorescein succinimidyl ester (CFSE) dilution were assessed 12 h and 72 h later, respectively. The percentage of CD25+cells and of dividing cells is shown. (e) Flow-sortedin vitroactivated human CD4+CD25+cells were transfected with nonspecific (NS), p65 or Sam68 siRNAs. The surface CD25 expression was analysed at 72 h, and the percentage of CD25+cells is shown. Figure 4: The critical role of Sam68 in the expression of the CD25 gene in T cells. ( a ) Jurkat cells were transfected with nonspecific (NS) or three different Sam68-specific siRNAs. After 72 h, the knockdown of Sam68 was examined by immunoblot (IB) for Sam68 with β-actin as a loading control. ( b ) NF-κB luciferase assay (mean±s.d., n =3) of Jurkat cells transfected with nonspecific (NS) or Sam68 siRNAs, together with indicated amount of p65 plasmids and a luciferase reporter gene driven by 5 × CD25 κB sites. ( c ) Real-time PCR quantization (mean±s.d., n =3) of mRNA level of CD25 normalized to GAPDH in Jurkat cells silenced with NS or pooled Sam68 siRNAs and stimulated by 50 ng ml −1 PMA plus 1.5 μM ionomycin (PMA/I) for indicated time. ( d ) Human peripheral blood T lymphocytes were transfected with nonspecific (NS), p65, or Sam68 siRNAs and then stimulated with PMA/I or left unstimulated (Unstim). Flow cytometry histograms of T cells with CD25 induction and carboxyfluorescein succinimidyl ester (CFSE) dilution were assessed 12 h and 72 h later, respectively. The percentage of CD25 + cells and of dividing cells is shown. ( e ) Flow-sorted in vitro activated human CD4 + CD25 + cells were transfected with nonspecific (NS), p65 or Sam68 siRNAs. The surface CD25 expression was analysed at 72 h, and the percentage of CD25 + cells is shown. Full size image CD25, a transmembrane protein, is critical for haematological cells to achieve a high-affinity binding of IL-2 (ref. 1 ). TCR engagement causes resting human T lymphocytes to transcriptionally upregulate several activation/proliferation mediators, in particular CD25 whose inducible expression depends on p65 but not RPS3 (ref. 7 ). Interestingly, knockdown of either Sam68 or p65, compared with nonspecific scramble siRNA oligonucleotides, retarded the PMA/I- or TCR engagement-induced CD25 induction in human T lymphocytes ( Fig. 4d and Supplementary Fig. S7 ). Consequently, attenuated cell surface CD25 expression due to Sam68 or p65 knockdown impaired TCR-induced human T lymphocyte proliferation ( Fig. 4d ). We further examined whether Sam68 is required to maintain the elevated CD25 in lymphocytes by transfecting siRNAs into activated human CD4 + CD25 + cells. As expected, nonspecific siRNA-silenced cells still maintained high surface CD25 expression ( Fig. 4e ). In contrast, Sam68 knockdown markedly attenuated surface CD25 expression, to a similar extent as p65 knockdown [7] ( Fig. 4e ). Together these results indicate that Sam68 is an important component of the CD25 NF-κB complex in both resting and activated T lymphocytes. To assess the impact of Sam68 on the TCR engagement-induced NF-κB gene transcription, which is critical for lymphocyte activation and proliferation [7] , [43] , [44] , we examined the effect of Sam68 knockdown on the induction of a subset of NF-κB genes in Jurkat cells. Compared with nonspecific scramble siRNA-transfected cells, Sam68 knockdown significantly attenuated the TCR stimulation-induced CD25 , BIRC3 , NFKB2 and CD83 genes ( Supplementary Fig. S8 ). In contrast, Sam68 knockdown augmented the BIRC2 and IL8 gene expression, and had no effect on the induction of CCL1 , USP12 , NFKBIA and TNFAIP3 genes ( Supplementary Fig. S8 ). Analogous with RPS3, as we reported previously [7] , [8] , Sam68 appears to control transcription of a selective subset of NF-κB target genes, in line with the evidence that it was only detected in a fraction of NF-κB DNA-binding complexes ( Fig. 2e ). Sam68 does not function as an adaptor in TCR signalling Containing several consensus domains to interact with SH3 domain-containing proteins and tyrosine kinases, Sam68 was proposed to function as an adaptor protein in lymphocyte activation signalling [19] , [34] . Moreover, Sam68 was recently shown to participate in the TNF signalling pathway [31] . We thus tested whether it functions as a signalling adaptor in TCR engagement-induced NF-κB signalling. We first verified that the Sam68 expression was not regulated during T-cell activation ( Fig. 5a and Supplementary Fig. S9 ). The CD3/CD28 antibodies and PMA/I-induced IκBα degradation in Jurkat cells with Sam68 knockdown was identical, if not more dramatic, to that in the cells transfected with nonspecific siRNA ( Fig. 5a ). Moreover, PMA/I induced an identical portion of p65 translocation from the cytosol to the nucleus in the control and Sam68 knockdown Jurkat cells ( Fig. 5b ). We further verified this result by immunofluorescence staining of p65 in Jurkat cells ( Fig. 5c ), and our quantified results showed that PMA/I triggered a significant p65 nuclear translocation in Sam68 knockdown cells, similar to the control cells ( Fig. 5d ). Together all these results demonstrate that Sam68 is not essential for the TCR engagement-initiated cytoplasmic signalling, which suggests that Sam68 most likely does not function as an adaptor molecule for TCR stimulation-induced NF-κB signalling. 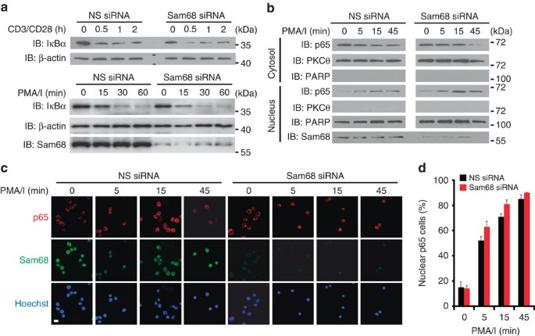Figure 5: Knockdown of Sam68 does not impair the TCR engagement-induced NF-κB signalling and p65 nuclear translocation. (a) Jurkat cells expressing either nonspecific (NS) or Sam68-specific siRNA were stimulated with anti-CD3/CD28 (1 μg ml−1each, top panel) or 50 ng ml−1PMA plus 1.5 μM ionomycin (PMA/I, bottom panel) for indicated periods. Whole-cell lysates were extracted and immunoblotted (IB) for IκBα and Sam68, with β-actin as a loading control. (b) Immunoblots using indicated antibodies of cytosolic and nuclear fractions derived from Jurkat cells transfected with indicated siRNAs and left unstimulated or stimulated with PMA/I for indicated periods. PKCθ and PARP served as cytosolic and nuclear markers, respectively. (c) Confocal micrographs of Jurkat cells silenced and stimulated as inb. The fixed cells were stained for Sam68, p65, and nuclei. (d) Percentage (mean±s.d.,n=3) of Jurkat cells (n>200) with nuclear p65 with nonspecific or Sam68-specific siRNA expression was quantified. Figure 5: Knockdown of Sam68 does not impair the TCR engagement-induced NF-κB signalling and p65 nuclear translocation. ( a ) Jurkat cells expressing either nonspecific (NS) or Sam68-specific siRNA were stimulated with anti-CD3/CD28 (1 μg ml −1 each, top panel) or 50 ng ml −1 PMA plus 1.5 μM ionomycin (PMA/I, bottom panel) for indicated periods. Whole-cell lysates were extracted and immunoblotted (IB) for IκBα and Sam68, with β-actin as a loading control. ( b ) Immunoblots using indicated antibodies of cytosolic and nuclear fractions derived from Jurkat cells transfected with indicated siRNAs and left unstimulated or stimulated with PMA/I for indicated periods. PKCθ and PARP served as cytosolic and nuclear markers, respectively. ( c ) Confocal micrographs of Jurkat cells silenced and stimulated as in b . The fixed cells were stained for Sam68, p65, and nuclei. ( d ) Percentage (mean±s.d., n =3) of Jurkat cells ( n >200) with nuclear p65 with nonspecific or Sam68-specific siRNA expression was quantified. Full size image Sam68 is phosphorylated by IKKα in the nucleus Sam68 appeared to not be associated with p65 in resting Jurkat cells; however, they complexed in the nucleus upon stimulation ( Supplementary Fig. S10 ), indicating an inducible interaction between Sam68 and p65 during T-cell activation. To understand how Sam68 participates in the NF-κB complex for CD25 gene transcription, we explored the post-translational modulation(s) of Sam68 during TCR engagement-induced NF-κB activation. Phosphorylation of Sam68 was previously shown to be critical for its nucleic acid-binding activity [19] , [24] , which led us to examine Sam68 phosphorylation during NF-κB activation. Our results revealed that Sam68 was phosphorylated at certain serine residue(s) in the nucleus following PMA/I stimulation ( Fig. 6a ). The IKK complex is an important group of serine/threonine kinases in NF-κB activation, which mainly consists of a regulatory subunit IKKγ and two catalytic subunits, IKKα and IKKβ (refs 4 , 5 ). Among them, IKKβ is almost an entirely cytoplasmic protein, whereas IKKα possesses a nuclear localization sequence (NLS) [4] , [5] that permits its nuclear translocation for NF-κB-dependent gene transcription [45] , [46] . In line with these findings, we observed a dramatic nuclear translocation of IKKα, in contrast to a modest nuclear accumulation of IKKβ in stimulated Jurkat cells, as shown by subcellular fractionation ( Fig. 6b ) and immunofluorescence microscopy ( Fig. 6c ). Moreover, Sam68, which preferentially localizes in the nucleus, did not appear to move from the cytoplasm in response to stimulation ( Fig. 5b ), thus apparently ruling out the possibility that IKKβ could phosphorylate Sam68 in the cytoplasm. Furthermore, the Sam68 serine-phosphorylation occurred in parallel with increased IKKα nuclear accumulation in activated Jurkat cells ( Fig. 6a ), hinting that IKKα could phosphorylate Sam68 in the nucleus. In support of this notion, IKKα as well as its active form was detected in the nucleus of HUT102 cells with high CD25 expression, but not Jurkat cells with low levels of surface CD25 ( Supplementary Fig. S11 ). Together these results suggest a potential link between IKKα nuclear translocation and CD25 expression via the phosphorylation of Sam68. 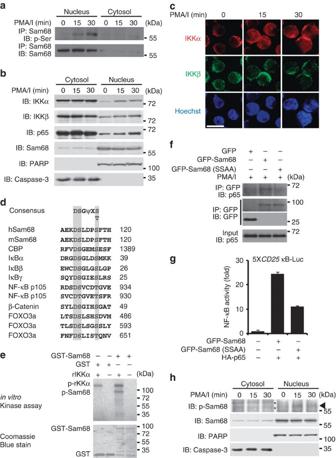Figure 6: IKKα phosphorylates Sam68 in the nucleus during TCR engagement-induced NF-κB activation. (a) Jurkat cells stimulated with PMA/I for indicated periods were fractionated into cytosolic and nuclear subcellular fractions, and then analysed by immunoprecipitation (IP) and immunoblotted (IB) with antibodies specific for Sam68 and serine-phosphorylated proteins (p-Ser). (b) Cytosolic and nuclear fractions derived from Jurkat cells stimulated as indicated were directly immunoblotted (IB) for indicated proteins. Full-length caspase 3 and PARP served as cytosolic and nuclear markers, respectively. (c) Confocal micrographs of Jurkat cells stimulated as indicated, and the fixed cells were stained for IKKα, IKKβ and nuclei. (d) Consensus motif of IKK phosphorylation sites. The sequence of Sam68 is aligned with those of CBP, IκBs, and other known substrates for comparison. The conserved phosphorylation motif for IKK is highlighted in grey (ψ, hydrophobic amino acid; X, any amino acid). The numbers at right show the position in the amino-acid sequence of the last residues depicted. (e) Autoradiograph (upper panel) and Coomassie blue-stained gel (bottom panel) ofin vitrokinase assays performed with recombinant GST or GST-Sam68 protein using recombinant human IKKα as kinase. The phosphorylated IKKα and Sam68 were labelled, respectively. (f) Whole-cell lysates from Jurkat cells expressing either GFP vehicle or indicated GFP-fused wild-type or mutant Sam68, were stimulated with PMA/I for 30 min and immunoblotted (IB) directly or after immunoprecipitation (IP) with GFP antibody for indicated proteins. (g) NF-κB luciferase assay (mean±s.d.,n=3) of Jurkat cells transfected with p65 and indicated GFP-fused wild type or mutant Sam68 plasmids together with a luciferase reporter gene driven by 5 ×CD25κB sites. (h) Cytosolic and nuclear fractions derived from Jurkat cells stimulated as indicated were directly immunoblotted (IB) for Sam68 phosphorylation with antibodies specific for S113/S117 phosphorylated Sam68 and general Sam68. Full-length Caspase 3 and PARP served as cytosolic and nuclear markers, respectively. Phosphorylated Sam68 is labelled by a triangle, and asterisks label nonspecific bands. Figure 6: IKKα phosphorylates Sam68 in the nucleus during TCR engagement-induced NF-κB activation. ( a ) Jurkat cells stimulated with PMA/I for indicated periods were fractionated into cytosolic and nuclear subcellular fractions, and then analysed by immunoprecipitation (IP) and immunoblotted (IB) with antibodies specific for Sam68 and serine-phosphorylated proteins (p-Ser). ( b ) Cytosolic and nuclear fractions derived from Jurkat cells stimulated as indicated were directly immunoblotted (IB) for indicated proteins. Full-length caspase 3 and PARP served as cytosolic and nuclear markers, respectively. ( c ) Confocal micrographs of Jurkat cells stimulated as indicated, and the fixed cells were stained for IKKα, IKKβ and nuclei. ( d ) Consensus motif of IKK phosphorylation sites. The sequence of Sam68 is aligned with those of CBP, IκBs, and other known substrates for comparison. The conserved phosphorylation motif for IKK is highlighted in grey (ψ, hydrophobic amino acid; X, any amino acid). The numbers at right show the position in the amino-acid sequence of the last residues depicted. ( e ) Autoradiograph (upper panel) and Coomassie blue-stained gel (bottom panel) of in vitro kinase assays performed with recombinant GST or GST-Sam68 protein using recombinant human IKKα as kinase. The phosphorylated IKKα and Sam68 were labelled, respectively. ( f ) Whole-cell lysates from Jurkat cells expressing either GFP vehicle or indicated GFP-fused wild-type or mutant Sam68, were stimulated with PMA/I for 30 min and immunoblotted (IB) directly or after immunoprecipitation (IP) with GFP antibody for indicated proteins. ( g ) NF-κB luciferase assay (mean±s.d., n =3) of Jurkat cells transfected with p65 and indicated GFP-fused wild type or mutant Sam68 plasmids together with a luciferase reporter gene driven by 5 × CD25 κB sites. ( h ) Cytosolic and nuclear fractions derived from Jurkat cells stimulated as indicated were directly immunoblotted (IB) for Sam68 phosphorylation with antibodies specific for S113/S117 phosphorylated Sam68 and general Sam68. Full-length Caspase 3 and PARP served as cytosolic and nuclear markers, respectively. Phosphorylated Sam68 is labelled by a triangle, and asterisks label nonspecific bands. Full size image By sequence alignment, a region within Sam68 (a.a. 112–117) was revealed to be similar to the characterized IKK consensus motif, DpSGΨXpS/T [4] ( Fig. 6d ). We therefore examined whether Sam68 could be a novel substrate of IKKα by an in vitro kinase assay. Besides autophosphorylation, recombinant IKKα strongly phosphorylated GST-Sam68, but not GST control ( Fig. 6e ), indicating that Sam68 is an IKKα substrate. To address the importance of serines 113 and 117 (S113/S117) phosphorylation for Sam68′s function in NF-κB signalling, we generated a S113A/S117A (SSAA) mutant Sam68 with the serines substituted with alanines, and examined the association of Sam68 to p65 and its ability to drive the CD25 κB site-luciferase reporter expression. The p65–Sam68 interaction was substantially attenuated by the alanine substitution in the stimulated Jurkat cells ( Fig. 6f ). This result suggests that the S113/S117 phosphorylation is critical for Sam68 to associate with p65, in line with the induced Sam68–p65 interaction during T-cell activation ( Supplementary Fig. S10 ). Moreover, ectopic expression of wild-type Sam68, together with p65, induced the CD25 κB-driven luciferase reporter expression. By contrast, the SSAA mutant Sam68 overexpression induced luciferase reporter gene expression was reduced 55%, compared with the wild-type Sam68 ( Fig. 6g ), suggesting that the alanine substitution dampens the Sam68- and p65-dependent CD25 reporter gene transactivation. Similarly, the induction of the CD25 κB luciferase reporter gene by overexpression of p65 with the ΔKH truncated Sam68, another mutant with diminished interaction with p65 ( Fig. 3d ), was also markedly attenuated ( Supplementary Fig. S12 ). Our results hence suggest that the S113/S117 phosphorylation is key for the Sam68–p65 association and its conferred CD25 gene transcription. To examine whether endogenous Sam68 was phosphorylated by IKKα, we generated an antibody that recognizes the S113/S117 phosphorylated form of Sam68. Indeed, we confirmed that endogenous Sam68 was S113/S117 phosphorylated in a time-dependent manner upon TCR activation in Jurkat cells ( Fig. 6h ). Thus, our results illustrate the serine phosphorylation of Sam68 by IKKα in the nucleus is critical for the NF-κB-mediated selective transcription of the CD25 gene, thus adding a new layer of specificity to the TCR-induced NF-κB activation. Sam68 is involved in various cellular processes including signal transduction, transcription, RNA metabolism, cell cycle regulation and apoptosis [19] , [20] , however, its physiological role, especially in lymphocyte activation has been enigmatic. Emerging evidence implicates that Sam68 has a critical role in transcriptional regulation. Specifically, Sam68 binds to hnRNP K and subsequently inhibits the latter’s function in transactivation of c-Myc target genes [32] . Moreover, Sam68 was proposed to function as a transcriptional coregulator to enhance the transcriptional activity of the androgen receptor and mixed lineage leukaemia complex [33] , [34] . Here we show that Sam68 is recruited to the CD25 promoter and facilitates p65 binding to CD25 κB DNA in normal and transformed human T cells, suggesting a novel role of Sam68 in NF-κB gene regulation. More importantly, we now discovered a major physiological role for Sam68 in human lymphocyte activation. Of note, our preliminary study indicates that Sam68 appears dispensable for receptor engagement-induced CD25 expression in mouse T cells. The different requirement for Sam68 in the CD25 promoter recognition could be due to the distinct usage of the NF-κB Rel components to initiate CD25 gene transactivation in human versus mouse T cells. The p65 and p50 subunits are the major NF-κB Rel components in the CD25 κB DNA-binding complex in normal and transformed human T cells ( Figs 1c , 2e and 3b ), and knockdown of Sam68 markedly impairs the CD25 upregulation, cell activation and proliferation in human T cells ( Fig. 4c–e ). In contrast, c-Rel was proposed to be the key NF-κB subunit supporting CD25 gene expression in mouse T cells [47] , [48] . Hence our results reveal an important role of Sam68 in regulating human T-cell signalling and CD25 expression. The function of Sam68 in mice and the distinct roles of Sam68 in human and mouse T-cell signalling are certainly worth further investigation. The IKK complex contains three major components: catalytic subunits IKKα and IKKβ and regulatory subunit IKKγ [4] , [49] . IKKβ is the major kinase that phosphorylates IκBα and appears to be almost an entirely cytoplasmic protein [4] , [50] ; whereas recent studies demonstrate that IKKα can enter the nucleus with a functional NLS [51] . The nuclear IKKα has been thought to largely remove negative regulators of NF-κB-dependent gene transcription by phosphorylating the transcriptional repressor complex [52] , chromatin-bound p65 (ref. 53 ), or CREB-binding protein [46] . Strikingly, IKKα was shown to be recruited, together with p65, onto NF-κB target gene promoters where IKKα-mediated phosphorylation of histone H3 thus modulates chromatin accessibility [45] , [54] . More recently, a promoter-specific function of IKKα in the nucleus was highlighted by the finding that nuclear IKKα was required for p65 DNA binding in a gene-specific manner albeit with no involvement of the histone H3 modification [55] . Here we demonstrated Sam68, a preferentially nuclear protein, is a novel substrate of IKKα. Therefore, IKKα appears to have a more sophisticated role in specifying NF-κB transcription by modulating multiple proteins in the nucleus. CD25 has a significant role in both hematopoietic malignancies and solid tumours [2] . CD25 expression and aberrant NF-κB signalling in the tumours themselves can lead to increased proliferation, anti-apoptotic protein expression and drug resistance. Monoclonal antibodies against CD25 are a significant treatment for patients with CD25-expressed cancers [56] ; however, inadequate delivery of the antibody directly to the tumour site may still be problematic, especially in patients with solid tumours expressing CD25. Sam68, a non-Rel component of NF-κB that confers CD25 gene transcription, could be a novel target for pharmacological interventions. Small molecule inhibitors targeting the p65–Sam68 association may be used to extinguish CD25 expression, in particular, in tumours that depend on CD25 for survival. Cells and reagents Jurkat E6.1, CEM, MT-2, HEK293T (purchased from ATCC) and HUT102 (kindly provided by T. Waldmann at NCI) cells were cultured in RPMI 1640 medium containing 10% fetal calf serum, 2 mM glutamine, and 100 U/ml each of penicillin and streptomycin. Human peripheral blood lymphocytes were isolated from healthy donor blood as previously described [7] . Antibodies used were: p65, p50, Sam68, IκBα (Santa Cruz); β-actin, FLAG, and HA (Sigma); CD25, Caspase3, IKKα, IKKβ and PARP (BD); phospho-Serine (Millipore); MYC and PKCθ (Cell Signaling) and GFP (Roche). RPS3 rabbit antibody was as described [7] . The rabbit polyclonal antibody specific for S113 and S117 phosphorylated Sam68 was generated and affinity purified using the peptide NH 2 -CAEKD(Sp)LDP(Sp)FTH-COOH by Primm (Cambridge, MA). Recombinant p65 and p50 proteins were purchased from Active Motif Inc. Plasmid constructs The pEGFP-p65 as well as various p65 truncation constructs, and pGEX-Sam68, pMYC-Sam68, pEGFP-Sam68 as well as various Sam68 truncation constructs were described previously [7] , [57] . The SSAA mutant of Sam68 was generated by site-directed mutagenesis using the Quick Change Kit (Stratagene) with appropriate primers for S113A/S117A, and verified by DNA sequencing. RNA interference and transfection The siRNA (sense-strand sequence) Sam68-duplex1, 5′-CCUGCACCAGAAACAUACGAAGAUU-3′; Sam68-duplex2, 5′-GAGAGCAUCCAUAUGGACGUUAUUA-3′; Sam68-duplex3, 5′-GAGACUGGUGCAAAGAUCUCUGUAU-3′ (Life Technologies). CD25 pool siRNA was purchased from Santa Cruz. The siRNA sequences for human RPS3 and p65 have been described [7] . Transient transfection of siRNA and/or DNA constructs into Jurkat cells, HEK293T cells, resting and activated human peripheral blood lymphocytes were performed as described previously [7] . Subcellular fractionation and DNA affinity purification Subcellular fractionation was performed by differential centrifugation as described [7] . In brief, cells were resuspended in ice-cold Buffer A (10 mM HEPES pH 7.9, 10 mM KCl, 1.5 mM MgCl 2 , 0.1 mM EDTA, 0.5 mM DTT, 0.4% NP-40, 0.5 mM PMSF, 1 × complete protease inhibitor cocktail (Roche)). Pellets were incubated in Buffer C (20 mM HEPES pH 7.9, 420 mM NaCl, 1.5 mM MgCl 2 , 25% glycerol, 0.5 mM PMSF, 0.2 mM EDTA, 0.5 mM DTT, 1 × complete protease inhibitor cocktail). The nuclear extract from HUT102 cells was adjusted to 20 mM HEPES buffer (pH 7.9) containing 150 mM NaCl, 10% glycerol, 0.5 mM DTT, 0.2 mM EDTA, 0.5 mM PMSF, 0.5 mM MgCl 2 and fractionated on Superose 6 column (GE Healthcare) by gel filtration chromatography. Fractions were separated by SDS–PAGE followed by western blotting or assayed for specific CD25 κB DNA-binding activity using EMSAs. Active fractions (24–28) were pooled and then further purified by DNA affinity. Following a preincubation with 30 mg ml −1 poly(dI-dC) competitor DNA, protein fractions were further purified with biotin-labelled vehicle oligonucleotides or double-stranded DNA containing five copies of CD25 κB sites and Streptavidin Sepharose (GE Healthcare) at 4 °C with gentle agitation for 2 h. The affinity-purified polypeptides were electrophoresed on SDS–PAGE followed by western blotting. Luciferase reporter gene assays Luciferase reporter gene assays were performed as previously described [7] . Briefly, cells were cotransfected at a ratio of 10:1 with various promoter-driven firefly luciferase constructs to the renilla luciferase pTKRL plasmid, together with indicated cDNA under some conditions. Cells were cultured for 1–2 days and then stimulated in triplicate before harvest. Lysates were analysed using the Dual-Luciferase Kit (Promega). Chromatin immunoprecipitation (ChIP) ChIP assays were performed as described [7] . The following primers were used to amplify the promoter region adjacent to the corresponding κB site: human CD25 promoter (−437 to −234): 5′-GAATATTGGAGGCTGCCTGA-3′ and 5′-TCAGCTACGCCCATAAAAGG-3′ (ref. 58 ), human NFKBIA promoter (−316 to −15): 5′-GACGACCCCAATTCAAATCG-3′ and 5′-TCAGGCTCGGGGAATTTCC-3′; human IL8 promoter (−121 to +61): 5′-GGGCCATCAGTTGCAAATC-3′ and 5′-TTCCTTCCGGTGGTTTCTTC-3′; and human ACTB promoter (−980 to −915): 5′-TGCACTGTGCGGCGAAGC-3′ and 5′-TCGAGCCATAAAAGGCAA-3′ (ref. 7 ). Electrophoretic mobility shift assays (EMSAs) EMSAs were carried out as described [7] , [59] . Double-stranded oligonucleotide probes (sense strand shown) used were NFKBIA -κB, 5′-CTGGTCGGAAGGACTTTCCAGCCAC-3′; CD25 -κB, 5′-CGGCAGGGGAATCTCCCTCTCC-3′. Samples were resolved on 6% DNA retardation gel (Life Technologies) in 0.25 × TBE buffer, and autoradiography was carried out on dried gels. Immunofluorescence microscopy Confocal microscopy was performed as previously described [7] . Briefly, cells were fixed with 4% paraformaldehyde in PBS and then Cellspin mounted onto slides. After a 5-min permeabilization with 0.05% Triton X-100 in PBS, the fixed cells were stained with appropriate primary antibodies for 45 min, and FITC- or AlexaFluor 594-conjugated secondary antibodies (Life Technologies) for 45 min together with 1 μg ml −1 of Hoechst 33342 (Sigma) for 5 min at 25 °C. The slides were then rinsed with PBS three times and cover mounted for fluorescence microscopy. Immunoprecipitation and western blot The cells were harvested and lysed on ice by 0.4 ml of TNTG lysis buffer (30 mM Tris–HCl (pH 8.0), 150 mM NaCl, 1% Triton X-100, and 10% glycerol, 1 × complete protease inhibitor cocktail) for 30 min. The lysates were centrifuged at 10,000 × g at 4 °C for 10 min. The protein-normalized lysates were subjected to immunoprecipitation by adding 10 mg ml −1 of the appropriate antibody, 30 μl of protein G-agarose (Roche), and rotating for more than 2 h in the cold room. The precipitates were washed at least five times with cold TNTG lysis buffer followed by a separation by SDS–PAGE under reduced and denaturing conditions. The resolved protein bands were transferred onto nitrocellulose membranes, probed as described previously [7] , [58] and developed by the Super Signaling system (Pierce, Rockford, IL) according to the manufacturer's instructions. Real-time PCR The RNA isolation and cDNA preparation were as described [7] . Real-time PCR reactions were performed in triplicate using the SYBR Green PCR Master Mix (Applied Biosystems) in a 7900HT sequence detection system (Applied Biosystems) with the following primers: GAPDH -f, 5′-CACATCAAGAAGGTGGTG-3′; and GAPDH -r, 5′-TGTCATACCAGGAAATGA-3′; CD25 -f, 5′-CCAGAGATCCCACACGCCACATTCAAAG-3′; and CD25 -r, 5′-GCATTGACATTGGTTGTCCCAGGACGAG-3′. The relative transcription level was calculated using the ΔΔCt method. In vitro kinase assay Kinase-active recombinant IKKα protein was purchased from Millipore (Billerica, MA). Bacterially purified glutathione S-transferase (GST) and GST-Sam68 were used as substrates. In vitro kinase assay was performed as described [11] . Briefly, enzyme (100 ng) and substrate (2 μg) were incubated in reaction buffer (25 mM Tris–HCl (pH 8.0), 50 mM KCl, 10 mM MgCl 2 , 1 mM DTT, 1 mM Na 3 VO 4 , 1 mM ATP) with 0.5 μCi 32 P-γ-ATP (GE Healthcare) added at 37 °C for 30 min. The reactions were resolved by SDS–PAGE and visualized by autoradiography. How to cite this article: Fu, K. et al . Sam68 modulates the promoter specificity of NF-κB and mediates expression of CD25 in activated T cells. Nat. Commun. 4:1909 doi: 10.1038/ncomms2916 (2013).